In vivocardiac phase response curve elucidates human respiratory heart rate variability Recovering interaction of endogenous rhythms from observations is challenging, especially if a mathematical model explaining the behaviour of the system is unknown. The decisive information for successful reconstruction of the dynamics is the sensitivity of an oscillator to external influences, which is quantified by its phase response curve. Here we present a technique that allows the extraction of the phase response curve from a non-invasive observation of a system consisting of two interacting oscillators—in this case heartbeat and respiration—in its natural environment and under free-running conditions. We use this method to obtain the phase-coupling functions describing cardiorespiratory interactions and the phase response curve of 17 healthy humans. We show for the first time the phase at which the cardiac beat is susceptible to respiratory drive and extract the respiratory-related component of heart rate variability. This non-invasive method for the determination of phase response curves of coupled oscillators may find application in many scientific disciplines. Since the observation of respiratory-related variation of the heart rate by S. Hales in 1733 and its first registration by C. Ludwig in 1847 (ref. 1 ), cardiorespiratory interaction (CRI) remains a challenging physiological phenomenon. Respiratory sinus arrhythmia as a component of heart rate variability has become important in many medical fields as a diagnostically and prognostically meaningful indicator of vagal activity. In a more general context, understanding interaction of oscillatory systems is a key problem for many areas of research, especially in life sciences, where rhythmical activity is both abundant and important. Many biological (sub)systems exhibit endogenous rhythms; quantification of their interaction with the environment is relevant for gaining insight into the orchestration of organismic processes, the dynamics of neuronal ensembles, determination of brain connectivity, study of robustness of circadian rhythms, and so on [2] , [3] , [4] , [5] , [6] . A key feature determining the interaction properties is the ability of an oscillator to respond, by shifting its phase, to an external perturbation; this feature is often quantified in terms of phase response curves (PRC), which describe both reactions to a single pulse perturbation and to a continuous force, resulting in a continuous phase shift in the latter case [2] , [3] , [7] , [8] . This approach is used in neuroscience [9] , [10] , [11] , cardiorespiratory physiology [12] , [13] , [14] , [15] , [16] , [17] and chronobiology [18] , [19] , to name just a few. A traditional experimental approach to obtain the PRC implies that the oscillator (for example, a neuron) is isolated from the environment (for example, from other neurons that normally interact with it) and is repeatedly perturbed by (weak) short pulses [20] . PRC is then defined as the phase shift evoked by the pulse; this shift is expressed as a function of the fraction of the oscillation period at which the pulse is applied. The aim of this Communication is two-fold: we present a new framework that allows us to reveal the PRC without isolating the system from its environment and without adding any specially designed perturbation, but from simple observation of the system and of the environment under free-running conditions, and to determine the PRC of human heartbeat in vivo. PRC is one of the basic concepts of nonlinear science [2] , [3] , [7] , [8] , universally applicable to endogenous, self-sustained oscillators (and clusters of oscillators [21] , [22] ) of various nature: physical, chemical, biological, and so on. The starting point here is a parametrization of the state of an isolated system with well-pronounced rhythmicity, for example, of an atrial pacemaker cell, by the phase φ . This uniformly growing variable measures the fraction of the time within one undisturbed cycle. An (not too strong) interaction with another endogenous oscillator can be characterized by the coupled dynamics of two phases φ 1 , φ 2 [7] : where ω 1,2 are natural, autonomous frequencies and q 1,2 are called the coupling (interaction) functions (Following the tradition of the physics literature, we understand coupling as the presence of an interaction between the oscillators, whereas in the biological literature coupling is often understood as a correlation between their outputs, for example, due to phase locking, cf. (refs 23 , 24 , 25 )). Equation (1) describes the ideal case when the two interacting oscillators are noise-free and are isolated from the rest of the world. If one goes beyond this ideal case, then the right-hand side of equation (1) contains additional terms, not related to the coupling, cf. equation (3) below. We stress that here we exploit the general concept of the phase from the dynamical systems theory. It characterizes relative accelerations/decelerations at different stages of the cycle; physiological (biological, physical, and so on) interpretation of phase values requires a separate consideration for any particular system. Theory [7] suggests that for weak interaction the coupling functions in typical cases can be written as where Z 1 ( φ 1 ) is the PRC of the first oscillator and I 2 ( φ 2 ) is the forcing with which the oscillator 2 acts on 1, and similarly for q 2 = Z 2 ( φ 2 ) I 1 ( φ 1 ). However, even if the governing equations for the interacting systems are known (like for many physical and engineering systems), the derivation of the phase model (1) and of the PRC represents a complicated theoretical problem. In this Communication, we develop a novel approach based on data analysis of free-running systems and demonstrate how the functions q , Z and I can be obtained non-invasively from observations of the coupled oscillatory systems in their natural environment. The advantage of using the phase model is its universal form. However, one cannot measure the phases directly; in fact only the time series of one or several observables of each oscillator are available. Typically, the phase is estimated from these time series [26] , [27] , [28] , [29] , but these estimates naturally depend on the observables and their processing. On the contrary, in the theory leading to equation (1), the phase is introduced in a unique way, as the variable that uniformly parametrizes the motion along the closed attractive curve in the state space of the dynamical system, that is, along the limit cycle. The gap between the theory and data-based model reconstruction can be bridged by means of the transformation of the initial phase estimate, called protophase, to the true phase, consistent with the theoretical definition [27] . This transformation ensures invariance of the model reconstruction and, hence, of the PRC determination for a large class of observables. We apply this approach for the first time to analyse the CRI in healthy humans, where we consider the heartbeat and the respiratory cycles as outputs of coupled oscillatory systems approximately obeying the description (1). From the observations of the electrocardiogram and arterial pulse and from the measurements of the respiration we first determine the true phases of these oscillators, then find the interaction function q , and finally determine the PRC Z and the forcing I . Human CRI has been studied for decades [23] , [24] , [25] , [30] , [31] , [32] , [33] . It has gained increased interest due to extensive application of ideas from nonlinear dynamics and information theory to medical problems, for example, to the use of heart rate variability (HRV) as an indicator of autonomic activity. As a result, many aspects of cardiorespiratory coordination, like the degree of locking and the directionality of interaction, have been investigated [26] , [28] , [29] , [34] , [35] , [36] , [37] , [38] , [39] , [40] . Here exploiting the invariant approach and the novel technique for the phase estimation of complex signals, we perform the evaluation of the coupling function and its decomposition into the PRC of the intact human heart and the respiratory forcing. Based on this, we quantify the respiratory-related component of the heart rate variability. This complete, from the viewpoint of the nonlinear dynamics theory, description of the phase dynamics of the CRI is promising for quantification of HRV. Coupling function and PRC from passive observation First we outline our framework ( Fig. 1 ) for the coupling function reconstruction ( cf. (refs 27 , 40 , 41 )) and the PRC determination from data. We emphasize the novel aspects of the procedure, whereas the details are described in Methods and Supplementary Information . 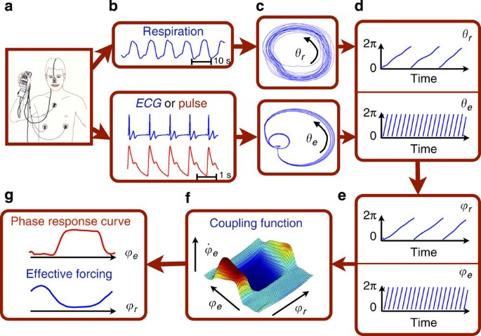Figure 1: Phase response curve from non-invasive observation: scheme of the approach. (a,b) The respiratory signal, the electrocardiogram, and the arterial pulse are simultaneously recorded from subjects in resting state. (c,d) From these scalar signals, by virtue of a proper 2D embedding, the protophasesθr,θe, andθpare obtained and transformed to the phasesφr,φe, andφp, shown ine. (In this schematic representation the difference betweenθeandφeis not seen). (f) The coupling (interaction) function describing the effect of respiration on heart dynamics is reconstructed in an invariant way. (g) The coupling function is decomposed into the phase response curve PRC and the respiratory forcing. Figure 1: Phase response curve from non-invasive observation: scheme of the approach. ( a , b ) The respiratory signal, the electrocardiogram, and the arterial pulse are simultaneously recorded from subjects in resting state. ( c , d ) From these scalar signals, by virtue of a proper 2D embedding, the protophases θ r , θ e , and θ p are obtained and transformed to the phases φ r , φ e , and φ p , shown in e . (In this schematic representation the difference between θ e and φ e is not seen). ( f ) The coupling (interaction) function describing the effect of respiration on heart dynamics is reconstructed in an invariant way. ( g ) The coupling function is decomposed into the phase response curve PRC and the respiratory forcing. Full size image The first step is to obtain high-resolution recordings of observables from two systems—one observable for the respiratory system and two different observables for the cardiovascular one: the ECG and the arterial pulse. The second step is parametrizing the signal by an angle variable θ that grows monotonically in time and gains 2π at each cycle. It is important that this variable, called protophase [27] , is unambiguously determined from the state of the oscillatory system. For complex waveforms like the ECG signal the construction of the protophase is highly non-trivial. Here we use a novel three-step technique: first we define six marker events within each cardiac cycle and introduce a preliminary cyclic variable from the conditions that it gains 2π between two R-peaks and linearly increases with time between the events. Next, we use this initial estimate to construct the average cycle and define a new, improved continuous protophase on it; finally, we assign the protophases to all points of the state plane trajectory by projecting them onto the average cycle. The protophase for the arterial pulse is obtained in a similar way, using 3 markers. The next step is to transform the protophases θ to phases φ , to match the underlying condition of equation (1) that the phase of an autonomous system grows uniformly in time. In this way an arbitrary protophase is mapped onto the uniquely defined phase; moreover, the transformation θ → φ is fully invertible and does not contain any filtering. Practically, it is performed by means of the probability distribution of θ , which is obtained by virtue of a kernel function [27] , [42] . Having two time series of the phases φ 1,2 , we represent their dynamics according to equation (1), via reconstructing the right-hand sides of equation (1) by virtue of two-dimensional (2D) kernel functions. We denote the phases from the ECG, the arterial pulse and the respiratory signal as φ e , φ p , and φ r , respectively. We reconstruct only the phase dynamics of the cardiac system, that is, only one of the equation (1); in the new notations it reads The residues of fitting ξ e,p ( t ) include noise and effects of non-observed physiological rhythms other than respiration, that is, ξ e,p describes all perturbations to the heart dynamics that do not depend on φ r . As the ECG and the arterial pulse represent two different observables of the cardiac system, ideally functions Q e ( φ e , φ r ), Q p ( φ p , φ r ) should coincide. In practice they are very similar in shape ( Fig. 2 ), which confirms the reliability of our approach and its invariance with respect to the used observables, due to the θ→ φ transformation. 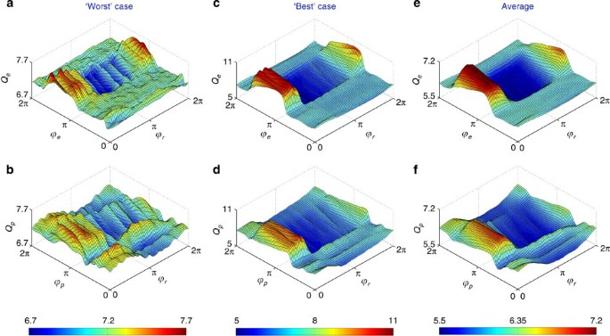Figure 2: Coupling functions for the human cardiorespiratory system. The reconstructed functions provide the dependence of the instantaneous cardiac frequency, measured in radians per second, on the cardiac and respiratory phases. Red regions mean higher frequencies (acceleration), whereas blue regions correspond to lower frequencies (deceleration). FunctionsQe(φe,φr) (a,c,e) are obtained from the ECG and the respiration, whereas functionsQp(φp,φr) (b,d,f) are computed from arterial pulse and respiration. Using these two very different observables for the cardiovascular system, we nevertheless obtain highly correlated results, as is expected for the invariant approach. The functions for the subject with the lowest correlation betweenQeandQpare shown in (a,b), and for the subject with the highest correlation in (c,d). Panels (e,f) present the averaged (over all measurements for all subjects) coupling functionsQeandQp. Figure 2: Coupling functions for the human cardiorespiratory system. The reconstructed functions provide the dependence of the instantaneous cardiac frequency, measured in radians per second, on the cardiac and respiratory phases. Red regions mean higher frequencies (acceleration), whereas blue regions correspond to lower frequencies (deceleration). Functions Q e ( φ e , φ r ) ( a , c , e ) are obtained from the ECG and the respiration, whereas functions Q p ( φ p , φ r ) ( b , d , f ) are computed from arterial pulse and respiration. Using these two very different observables for the cardiovascular system, we nevertheless obtain highly correlated results, as is expected for the invariant approach. The functions for the subject with the lowest correlation between Q e and Q p are shown in ( a , b ), and for the subject with the highest correlation in ( c , d ). Panels ( e , f ) present the averaged (over all measurements for all subjects) coupling functions Q e and Q p . Full size image The last stage is an optimal decomposition Q e,p ( φ e,p , φ r )=ω e,p + Z ( φ e,p ) I ( φ r )+β( φ e,p , φ r ), cf. equation (2), which minimizes the residual error β . We find that the error is relatively small; hence, the resulting functions Z ( φ e,p ) and I ( φ r ) can be interpreted, according to the theoretical framework, as the PRC and the driving force, respectively. Coupling function for cardiorespiratory interaction The intermediate result of our analysis, that is, the reconstructed coupling functions Q e,p ( φ e,p , φ r ), are illustrated in Fig. 2 . Before making the next step, we discuss the robustness of the obtained functions for different test persons and trials. The reliability of the technique is confirmed by large similarity between the coupling functions among the group, with highest similarity for repeated measurements of the same person. To quantify the similarity between the functions obtained in different trials, we use the correlation coefficient ρ , which quantifies similarity of the forms of two functions (independent on their amplitudes), and the difference measure η (see Methods ), which also reflects difference in the amplitudes (norms) (see Fig. 3 ). We find that the functions have a well-pronounced characteristic shape for each of the subjects ( Fig. 2e,f ): the correlations between Q e ( φ e , φ r ) obtained in different trials with the same subjects are ρ 0.6 (with the average ≈0.89). Naturally, the correlation between the functions of different subjects is lower, reflecting the interpersonal variability; however, it is high enough, ρ 0.43 (average ≈0.81), to demonstrate the high similarity of the CRI in our group of subjects. We emphasize that the high similarity of the functions, obtained from such different observables as the ECG and the arterial pulse, as well as practical coincidence of their norms, supports validity of the transformation to the invariant phase. 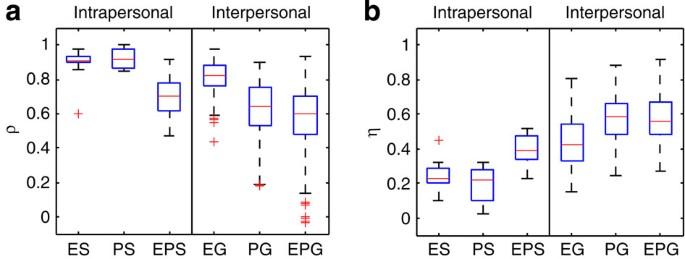Figure 3: Similarity measures for the obtained coupling fuctions. Box–whisker plot illustrates the correlation coefficientρ(a) and the difference measureη(b), for all available pairs of functions (high similarity corresponds to largeρand smallη). ES: similarity between the functionsQe(respiration—ECG) of the same subject, obtained from two trials; it is maximal. EG: similarity betweenQeof different subjects in the group demonstrates low interpersonal variability. PS and PG: intra- and interpersonal similarities forQp(respiration—arterial pulse). EPS and EPG: intra- and interpersonal similarities betweenQeandQp. Notice that the correlation can be maximized by computing it for phase-shifted functions; so, for example, the outlier value in (a) ES, at ≈0.6 becomes as high as 0.9. This phase-shift might reflect a variation of internal delays and therefore might have a physiological meaning; however, this issue requires a separate study. The number of cases used for computation of the six box plots is (from left to right): 11, 18, 29, 314, 172 and 491. (The low border of the box, the red line, and the upper border are the first, second and third quartiles, respectively. The whisker length is 1.5 times the interquartile range.) Figure 3: Similarity measures for the obtained coupling fuctions. Box–whisker plot illustrates the correlation coefficient ρ ( a ) and the difference measure η ( b ), for all available pairs of functions (high similarity corresponds to large ρ and small η ). ES: similarity between the functions Q e (respiration—ECG) of the same subject, obtained from two trials; it is maximal. EG: similarity between Q e of different subjects in the group demonstrates low interpersonal variability. PS and PG: intra- and interpersonal similarities for Q p (respiration—arterial pulse). EPS and EPG: intra- and interpersonal similarities between Q e and Q p . Notice that the correlation can be maximized by computing it for phase-shifted functions; so, for example, the outlier value in ( a ) ES, at ≈0.6 becomes as high as 0.9. This phase-shift might reflect a variation of internal delays and therefore might have a physiological meaning; however, this issue requires a separate study. The number of cases used for computation of the six box plots is (from left to right): 11, 18, 29, 314, 172 and 491. (The low border of the box, the red line, and the upper border are the first, second and third quartiles, respectively. The whisker length is 1.5 times the interquartile range.) Full size image We have also performed a surrogate data test [43] . First we computed two functions Q e for a subject, for whom data from two trials are available ( Fig. 4a,b ). Next, we used exactly the same procedure and computed two functions after interchanging the respiration time series from the trials ( Fig. 4c,d ). These surrogates keep the properties of the processes, but destroy the correlation between them. The functions shown in Fig. 4e,f are obtained by taking the respiration data of other subjects. Ideally, the functions obtained from the surrogate data should be flat, showing no coupling; in practice, we observe some low variability due to accidental phase correlations, because we have only 20–40 respiratory cycles. However, the difference measure η between the true and the surrogate functions is approximately one order in the magnitude larger than between the two true functions. We conclude that the detected coupling is not a statistical artefact; however, the surrogate tests do not allow one to check whether all components of the coupling are revealed. The absence of artefacts in the reconstructed function is also supported by numerical tests with artificial ECG signals. 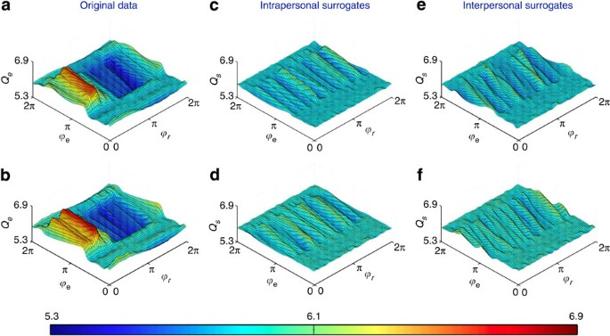Figure 4: Surrogate data test. Here we show an essential difference between true functionsQe(here for ECG-respiration) and spurious functionsQs. (a,b) Coupling functions for two recordings of the same subject (average heart rates are 0.93 Hz and 0.94 Hz, average respiration frequencies are 0.16 Hz and 0.13 Hz). (c,d) Coupling functions obtained after interchanging the respiratory signals from these two measurements. (e,f) Here respiration time series of a different subjects is used (average frequency 0.32). The difference measure,η, between the true functions (a) and (b) is 0.20, whereas the difference between the true function (a) and the spurious functions (c,e) is 0.81. The difference between (b) and its surrogates (d,f) is 0.80. The difference between the surrogates is in the range from 0.58 to 0.80. The correlation,ρ, between the true functions (a) and (b) is 0.93, whereas the correlation between the true function (a) and the spurious functions (c,e) is −0.10 and 0.00, respectively. The correlation between (b) and its surrogates (d,f) is 0.13 and 0.25. The absolute value of the correlation between the surrogates is in the range from 0.02 to 0.34. Figure 4: Surrogate data test. Here we show an essential difference between true functions Q e (here for ECG-respiration) and spurious functions Q s . ( a , b ) Coupling functions for two recordings of the same subject (average heart rates are 0.93 Hz and 0.94 Hz, average respiration frequencies are 0.16 Hz and 0.13 Hz). ( c , d ) Coupling functions obtained after interchanging the respiratory signals from these two measurements. ( e , f ) Here respiration time series of a different subjects is used (average frequency 0.32). The difference measure, η , between the true functions ( a ) and ( b ) is 0.20, whereas the difference between the true function ( a ) and the spurious functions ( c , e ) is 0.81. The difference between ( b ) and its surrogates ( d , f ) is 0.80. The difference between the surrogates is in the range from 0.58 to 0.80. The correlation, ρ , between the true functions ( a ) and ( b ) is 0.93, whereas the correlation between the true function ( a ) and the spurious functions ( c , e ) is −0.10 and 0.00, respectively. The correlation between ( b ) and its surrogates ( d , f ) is 0.13 and 0.25. The absolute value of the correlation between the surrogates is in the range from 0.02 to 0.34. Full size image PRC for cardiorespiratory interaction Final results for the computation of the PRC of the human heartbeat in vivo are presented in Fig. 5 . Below we restrict ourselves to the coupling functions obtained from the ECG data, as they are of superior quality; the results based on pulse time series are shown in Supplementary Fig. S1 . We show both the individual PRCs Z and the forcing functions I for all trials, as well as the group-averaged curves, obtained either by averaging all functions Z and all functions I , or by decomposing the averaged coupling function (shown in Fig. 2e ). As in the decomposition we cannot separately determine the amplitudes of the PRC and of the forcing, only the form of these functions is revealed (in our presentation in Fig. 5 we make the norms of Z and I equal, another option is illustrated in Supplementary Fig. S2 ). In Fig. 5c,d , we also show the relative decomposition errors, they all are in the range between 0.15 and 0.45, with median ≈0.265. 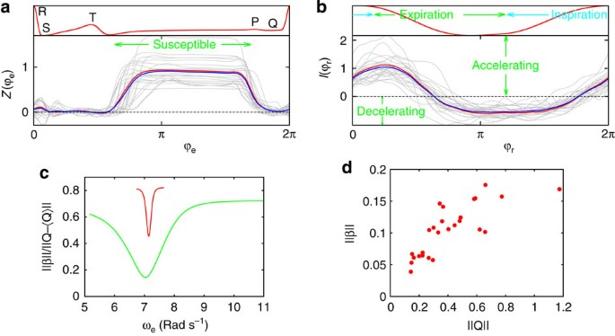Figure 5: PRC curves and effective forcing. We show individual PRCsZ(a) and effective forcingI(b) for all ECG-based coupling functions with grey curves. In both panels blue lines show the average over all individual (grey) curves. Red curves are obtained by decomposition of the averaged coupling function, shown inFig. 2e. Small panel on top of (a) shows for comparison the average ECG cycle as a function of its phase. One can clearly see the interval where PRC is not zero and, hence, the cardiac system is susceptible for the respiratory perturbation. Small panel on top of (b) shows the average respiratory cycle as a function of the phase, with marked epochs of inspiration and expiration (approximately). Intervals of positive (negative) effective forcing are the intervals where respiration is accelerating (decelerating) the heart rate. Panels (c,d) show error of the decomposition ||β||, where ||˙|| denotes the norm of the function. In (c) the relative erroris shown (for the cases of the largest (red) and of the smallest (green) error) in dependence on the parameterωeused in the decomposition procedure; finally the value ofωeyielding minimal error is chosen. In (d) all errors are presented, demonstrating quality of the decomposition. Figure 5: PRC curves and effective forcing. We show individual PRCs Z ( a ) and effective forcing I ( b ) for all ECG-based coupling functions with grey curves. In both panels blue lines show the average over all individual (grey) curves. Red curves are obtained by decomposition of the averaged coupling function, shown in Fig. 2e . Small panel on top of ( a ) shows for comparison the average ECG cycle as a function of its phase. One can clearly see the interval where PRC is not zero and, hence, the cardiac system is susceptible for the respiratory perturbation. Small panel on top of ( b ) shows the average respiratory cycle as a function of the phase, with marked epochs of inspiration and expiration (approximately). Intervals of positive (negative) effective forcing are the intervals where respiration is accelerating (decelerating) the heart rate. Panels ( c , d ) show error of the decomposition || β ||, where ||˙|| denotes the norm of the function. In ( c ) the relative error is shown (for the cases of the largest (red) and of the smallest (green) error) in dependence on the parameter ω e used in the decomposition procedure; finally the value of ω e yielding minimal error is chosen. In ( d ) all errors are presented, demonstrating quality of the decomposition. Full size image The PRC of the heartbeat, which is the main result of this study, clearly exhibits two different domains: in the interval 0.6π φ e 1.8π, the phase of the heartbeat can be strongly advanced by respiration forcing, and this susceptible epoch lies between the T and P waves. Another domain ( φ e 0.6π and φ e 1.8π) is characterized by nearly zero response, that is, here the heart is insensitive to respiratory drive. A corresponding interpretation for the respiratory force I follows from Fig. 5b . The functions I are quite close to a sine, but with a typical asymmetry of inspiration/expiration stages. As I changes sign (while Z is positive or close to zero), one can distinguish the different stages of accelerating and decelerating effects of force, and relate them to the stages of inspiration and expiration within the respiration cycle. Respiratory-related component of the heart rate variability Description of cardiorespiratory interaction in terms of coupling functions yields a new technique for the quantification of respiratory-related HRV. HRV is one of the central tools of psychophysiology and behavioural medicine [44] , and the respiratory component is a significant part of it [23] , [24] , [25] , [45] , [46] , [47] , [48] , representing mainly the vagal or parasympathetic part of the autonomic nervous system influences. Having introduced the time-continuous phase of the ECG, we obtain a continuous description of the HRV via the instantaneous frequency , instead of the commonly used discontinuous beat-to-beat description. Furthermore, using equation (3) we decompose into two processes: the first component, Q e ( φ e ( t ), φ r ( t )), reflects the effect of respiration and therefore can be used for characterization of the respiratory sinus arrhythmia (we use ‘RSA-HRV’ to denote this component), whereas the second component, ξ e ( t ), is independent of respiration and reflects both intrinsic sources of HRV as well as the effects of other unobserved rhythms like baroreflex and/or angiotensin loop rhythms and of random perturbations; we denote it as ‘non-RSA-HRV’ (Noteworthy, in 8 cases the RSA-HRV component is larger that non-RSA-HRV, and in 18 cases it is smaller, indicating, respectively, vagal and sympathetic predominance of the subjects during the measurements). The quality of this decomposition is confirmed by Fig. 6a : we see that the variances of the components sum up to the full variance of HRV, as is expected for independent components. This result, in addition to opening a new perspective in quantification of the respiratory influence on the heartbeat, provides a confirmation of our approach based on equation (3). 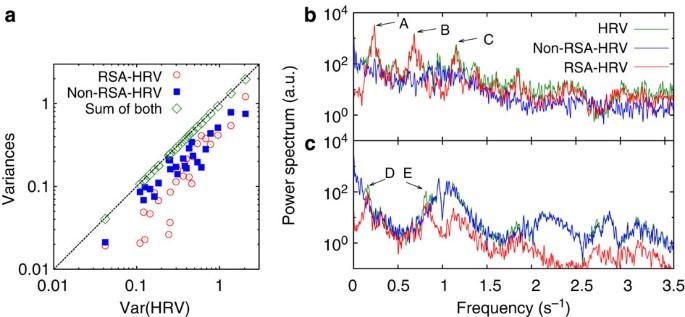Figure 6: Extracting the respiratory component of heart rate variability. (a) The variances of the RSA-HRV and non-RSA-HRV signals, as functions of the variance of the original HRV. Green diamonds show the sums Var(RSA-HRV)+Var(non-RSA-HRV), these are nearly equal to Var(HRV) (black dashed line), which means that RSA-HRV and non-RSA-HRV are almost uncorrelated. (b,c) Power spectra of original HRV (green), the RSA-HRV component (red) and of the non-RSA-HRV (blue), in the cases of maximal (b) and minimal (c) relative RSA-HRV component; in (b) ≈67% of Var(HRV) is contained in RSA-HRV, indicating vagal predominance, whereas in (c) only 10% Var(HRV) is in RSA-HRV, indicating sympathetic predominance. In (b) the letters A, B, C mark three respiratory-related peaks, corresponding to average respiratory frequency 0.23 Hz and to side-bands of the heart rate (average value 0.92 Hz), that is, to 0.92±0.23 Hz. Notice that these peaks (at which the green and red curves practically coincide) are definitely higher than the surrounding, which indicates a strong contribution of RSA-HRV in these frequency bands. Correspondingly, the residual non-RSA-HRV (blue line) is much weaker than HRV and RSA-HRV in these bands. Contrary, in (c) the peaks of RSA-HRV, marked by D (corresponds to average respiratory frequency 0.15 Hz) and E (side-band of the heart rate peak at ≈0.82 Hz) are low and the corresponding peaks in HRV only slightly exceed the surrounding; hence, the residual non-RSA-HRV is relatively high. Figure 6: Extracting the respiratory component of heart rate variability. ( a ) The variances of the RSA-HRV and non-RSA-HRV signals, as functions of the variance of the original HRV. Green diamonds show the sums Var(RSA-HRV)+Var(non-RSA-HRV), these are nearly equal to Var(HRV) (black dashed line), which means that RSA-HRV and non-RSA-HRV are almost uncorrelated. ( b , c ) Power spectra of original HRV (green), the RSA-HRV component (red) and of the non-RSA-HRV (blue), in the cases of maximal ( b ) and minimal ( c ) relative RSA-HRV component; in ( b ) ≈67% of Var(HRV) is contained in RSA-HRV, indicating vagal predominance, whereas in ( c ) only 10% Var(HRV) is in RSA-HRV, indicating sympathetic predominance. In ( b ) the letters A, B, C mark three respiratory-related peaks, corresponding to average respiratory frequency 0.23 Hz and to side-bands of the heart rate (average value 0.92 Hz), that is, to 0.92±0.23 Hz. Notice that these peaks (at which the green and red curves practically coincide) are definitely higher than the surrounding, which indicates a strong contribution of RSA-HRV in these frequency bands. Correspondingly, the residual non-RSA-HRV (blue line) is much weaker than HRV and RSA-HRV in these bands. Contrary, in ( c ) the peaks of RSA-HRV, marked by D (corresponds to average respiratory frequency 0.15 Hz) and E (side-band of the heart rate peak at ≈0.82 Hz) are low and the corresponding peaks in HRV only slightly exceed the surrounding; hence, the residual non-RSA-HRV is relatively high. Full size image To illustrate the decomposition in more detail, we show in Fig. 6b,c the power spectra of the original HRV and of their two components, for two extreme cases, that is, for maximum and minimum content of RSA-HRV in HRV, measured by the ratio rms(non-RSA-HRV)/rms(HRV). In both cases the main effect on the spectrum is elimination of a peak at the frequency of respiration (~0.2 Hz). Additionally, some respiration-induced side-bands close to the basic heart frequency are reduced, whereas the very low frequencies (<0.1 Hz) remain practically unchanged. We have presented a general framework for determination of PRC from the observations of coupled oscillators under free-running, undisturbed conditions, and have applied it to characterize the respiratory influence on the cardiac cycle in humans. Our reconstruction method is based solely on non-invasively recorded biological data and their analysis, and can be applied to a wide class of coupled self-sustained, endogenous systems, provided the oscillatory observables from both of them are available; the coupling should be not too strong, so that the oscillators remain asynchronous (presence/absence of synchrony can be easily recognized from the data). In our case the decomposition of the coupling function into a product of the PRC and the forcing was successful, which indicates that the interaction between the cardiovascular and the respiratory systems is relatively weak (in the sense of applicability of equation (1)). This allowed us for the first time to obtain the PRC of the heart in vivo and without artificial measures like paced breathing. Generally this decomposition may not work, so that the coupling function would be the final stage of the analysis. For a group of healthy subjects we have determined the functions describing the effective respiratory forcing, I , and the heart PRCs, Z , which, being multiplied, fully quantify the respiratory-related HRV. These functions provide a rather detailed, with a resolution much finer than the cycle length, description of the CRI on the system analysis level, without going into details of background chemical and electrical mechanisms. The functions I are quite close to a sine, but with a typical asymmetry of inspiration/expiration stages, which manifest itself in asymmetry of decelerating and accelerating stages of the forcing ( Fig. 5b ). On the contrary, the form of the PRC is highly non-sinusoidal and exhibits an epoch of insusceptibility, ≈40% of the cycle length (in phase units), where the PRC is close to zero and the heart is insensitive to forcing (in accordance to the known refractory period of sinoatrial cells [49] ). During the epoch of susceptibility, the phase of the heart can be influenced by the respiration, to our knowledge mainly by varying vagal control. This epoch coincides with the electrical diastole, that is, with the interval between T and P waves. This corresponds to the fact that in the second halve of the T-wave the cells of the myocardium recover and become again susceptible to excitation; this epoch is terminated with the next cycle of the sinus node activity, when atrial and ventricular excitation renders the myocardium refractory. The functions I and Z quantify the long known qualitative observation that inspiration accelerates the heartbeat, whereas expiration slows it down [50] and make it possible for the first time to determine, when these influences take place. It is well known [23] , [24] , [25] , [45] , [46] , [47] , [48] , [51] , [52] that the phase of respiration influences the peripheral autonomic nervous system’s outflow to the heart. However, till now it has never been shown when exactly this happens inside the cardiac cycle. Our results show that this transfer happens when the PRC is highest, that is, between T and P waves, which is the time of electrical diastole of the heart; they also correctly reveal the existence and timing of the atrial and ventricular refractory phase of the myocardium [49] , during which no information transfer takes place. This information is relevant for all models of CRI as well as for clinical problems (in particular because the period of susceptibility is crucial for myocardial fibrillation risk estimation). Our technique of non-invasive determination of refractory and susceptible periods is thus of potentially high medical and clinical relevance, as these periods demonstrate quite an interpersonal variability (see grey lines in Fig. 5a ). This information might be used to determine individual myocardial properties relevant for fibrillation. Furthermore, as the duration of electric diastole mainly determines the heart rate [53] , the amplitude of PRC can be considered as a measure of adaptability in response to respiratory drive; adaptation of the heart rate is a fundamental prerequisite of the proper functioning of the cardiovascular system. Therefore, quantification of variations of the PRC in amplitude or shape might be helpful for diagnostic of various disease states involving cardiorespiratory dysautonomia [54] . Further statistical studies of PRC dependence on the age, gender and other factors are needed here. In this paper we mainly concentrated on the reliability and consistency of the developed technique, which is confirmed by similar results obtained from ECG and arterial pulse, which are two essentially different observables of the same system, representing, respectively, electrical and mechanical processes in the heart. A further confirmation of the validity was achieved via a decomposition of the instantaneous frequency time series, which represents the HRV, into two components: the respiratory-related and the non-respiratory-related ones, which are found to be statistically independent. This fact indicates that the respiratory-induced part of HRV is correctly captured by our technique. Additionally, this essentially nonlinear decomposition opens new ways for quantification of the RSA and of the HRV, to be compared with other recently suggested decomposition methods based on linear analysis [55] , [56] . As the HRV analysis by itself has gained clinical relevance in fields like cardiac risk prognosis, sleep research and circadian autonomic regulation, we expect that our essentially nonlinear approach will contribute significantly to these studies, allowing one to go beyond a usual linear analysis. For our group of healthy subjects, the coupling functions and PRCs of the heart have a characteristic, reproducible shape, whereas the amplitude of these functions varies. This finding makes the approach promising for quantitative studies of possible effects of different factors (age, gender, diseases, drugs, physical load, and so on) on these characteristics of the cardiovascular physiology. To give a flavour of such possibilities, we show in Fig. 7 that the norms || Q || and, hence, the RSA-HRV tend to decrease with age, in good correspondence with other studies [57] , whereas the shape of Q does not exhibit an age dependence. However, clinical and physiological applications of cardiorespiratory coupling functions and PRCs require comprehensive statistical studies with different groups of subjects. Another prospective application of the characterization of CRI through PRC is related to implementation of a proper CRI in computational modelling of cardiac electrophysiology [58] . 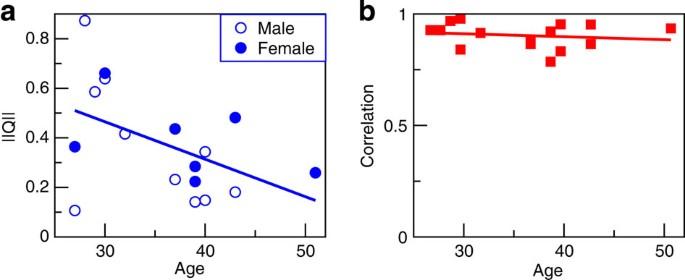Figure 7: Characterizing age dependence of cardiorespiratory interaction. (a) Age dependence of the norm of the coupling functionfor male (open circles) and female (filled circles) subjects shows that cardiorespiratory interaction tends to decrease with age (correlation coefficient is −0.48). Each symbol shows the average of norms of allQe,pcoupling functions available for one subject. (b) The correlation ofQewith the average function shown inFig. 2eversus the difference of the age and the average age (36 in our group) indicates independence of the shapeQon the age (correlation coefficient is −0.16). Figure 7: Characterizing age dependence of cardiorespiratory interaction. ( a ) Age dependence of the norm of the coupling function for male (open circles) and female (filled circles) subjects shows that cardiorespiratory interaction tends to decrease with age (correlation coefficient is −0.48). Each symbol shows the average of norms of all Q e,p coupling functions available for one subject. ( b ) The correlation of Q e with the average function shown in Fig. 2e versus the difference of the age and the average age (36 in our group) indicates independence of the shape Q on the age (correlation coefficient is −0.16). Full size image Data We analysed continuous multichannel recordings from 17 healthy subjects (7 females, 10 males; age between 27 and 51 years, average 36 years; see Supplementary Table S1 for details; written informed consent including permission of data use was obtained from all subjects before the measurement). The measurements were done with a custom-made battery-powered device (ChronoCord, Human Research Institute, Weiz, Austria ( www.humanresearch.at ) and FH Joanneum, Kapfenberg, Austria) with Bluetooth connection to a PC. It is based on a Holter ECG, but was expanded to record four channels, each with the sampling rate of 1 kHz and resolution of 16 bit. The device was equipped with a differential chest-wall ECG, two piezoresistive pressure sensors attached to the wrist of the left and right hands above the arteria radialis close to the location of apophysis radii and yielding arterial pulse signals, and a high-speed thermistor to record the nasal respiratory flow for the respiration signal [59] , [60] . For each subject, two recordings of duration 420 s were performed in the supine position at rest, with the interval of 12 min between the trials; the subjects were standing quietly and relaxed during these breaks. All data have been visually inspected and only time series without large disturbances, for example, due to motion, swallowing, and so on, were analysed (small artefacts have been manually corrected during preprocessing). Altogether, we have selected and analysed 26 records of respiration—ECG data and 20 records of respiration—arterial pulse data (see Supplementary Table S1 ). Preprocessing of time series has been performed in the following way: manual correction of artefacts by interpolation (for respiration), smoothing by Savitzky–Golay filter and elimination of slow baseline fluctuations (see Supplementary Figs S3–S5 ). Phases from data Protophases of the respiratory signal, θ r , were obtained as angles in the 2D embedding performed with help of the Hilbert Transform ( Fig. 8a ). Then, the protophases were transformed to the phases with the help of the technique of Kralemann et al . 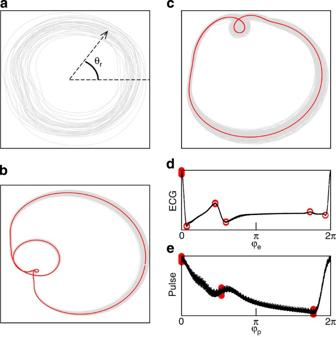Figure 8: Phase extraction from the registered data. 2D embeddings of the registered signals (grey lines) by virtue of the Hilbert transform (xcoordinate: original signal,ycoordinate: its Hilbert transform) for respiration (a) (here also the definition of the protophase is depicted), ECG (b), and arterial pulse (c). Red lines in (b,c) show the average cycles for the ECG and the arterial pulse. Panels (d,e) show marker events within one ECG cycle and arterial pulse cycle, respectively. [27] : Figure 8: Phase extraction from the registered data. 2D embeddings of the registered signals (grey lines) by virtue of the Hilbert transform ( x coordinate: original signal, y coordinate: its Hilbert transform) for respiration ( a ) (here also the definition of the protophase is depicted), ECG ( b ), and arterial pulse ( c ). Red lines in ( b , c ) show the average cycles for the ECG and the arterial pulse. Panels ( d , e ) show marker events within one ECG cycle and arterial pulse cycle, respectively. Full size image where are the coefficients of the Fourier expansion of the probability distribution density of θ , computed from its time series θ( t j ), where j =1,…, N . The number of Fourier modes n F was chosen according to the study by Tenreiro [42] . For such complex signals as ECG, the embedding via the Hilbert Transform does not provide a trajectory with a well-defined centre of rotation ( Fig. 8b ); therefore, we developed the following three-step technique. In the first step, six markers are identified within each PQRST complex, corresponding to the maxima of R, T and P waves and minima of Q, S and of the wave after T ( Fig. 8d ). The first estimate, Ψ, of the protophase is obtained by means of a linear interpolation between the markers, whereas the phase of each marker is assigned according to its average position within the cycle; the phase of the R-peak is set to zero. Next, we construct from the ECG the complex analytic signal z ( t ) by means of the Hilbert Transform, and compute the average cycle ( Fig. 8b ), parametrized by an angle variable ψ : where H n are the Fourier coefficients of the function z (ψ): As the next step we introduce the protophases θ e , projecting z ( t ) onto the average cycle with the help of an optimization strategy, illustrated in Supplementary Figs S6 and S7 . Finally, the transformation θ e → φ e was performed according to equation (4). The protophases θ p were obtained via the average cycle technique with 3 markers on the embedded cycle ( Fig. 8c ), see Fig. 8e . Coupling function reconstruction For this purpose we use the kernel density estimation. First, for each point in the data set we estimate the derivative of either φ e or φ p via local polynomial fitting, using the fourth-order Savitzky–Golay filter with the window length 0.008 s, which provided a reliable smoothing without losing much information. Next, we fit equation (3) on a n × n grid using the smoothing kernel with the width inverse proportional to n : . We compute Here φ e,p and φ r denote the points on the grid, where the functions Q e,p are estimated, whereas Φ e,p and Φ r denote the time series of cardiac and respiratory phases, respectively. We choose n =64 that yields ≈100 observation points per grid cell. Similarity between the functions is quantified by the correlation coefficient , which measures similarity of the forms of two functions (independently of their amplitudes), and by the difference measure , which also reflects difference in the amplitudes (norms). Here denotes averaging over the 2D domain 0 ≤ φ 1 , φ 2 ≤2π, , and norm . PRC from coupling function We decompose the reconstructed functions Q e ( φ e , φ r ) according to equation (3). As the frequency ω e is unknown, we represent Q e ( φ e , φ r )–ω e = Z ( φ e ) I ( φ r ) as a product of two functions, considering ω e as a parameter and searching for minimum of the decomposition error ; the optimal value is taken for the estimate of the frequency ω e (see Fig. 5c ). Decomposition of a function into a product was performed by means of an iterative scheme ( Supplementary Equation (S5) ). How to cite this article: Kralemann, B. et al . In vivo cardiac phase response curve elucidates human respiratory heart rate variability. Nat. Commun. 4:2418 doi: 10.1038/ncomms3418 (2013).